A polychromatic approach to far-field superlensing at visible wavelengths Breaking the diffraction barrier in the visible part of the electromagnetic spectrum is of fundamental importance. Far-field subwavelength focusing of light could, for instance, drastically broaden the possibilities available in nanolithography, light-matter interactions and sensing at the nanoscale. Similarly, imaging with a nanometric resolution could result in incredible breakthroughs in soft matter and biology. There have been numerous proposals in this regard based on metamaterials, structured illumination methods or diffractive optical components. The common denominator of all these approaches resides in their monochromatic nature. Here we show that using polychromatic light in dispersive metamaterials allows us to circumvent many limitations associated with previous monochromatic approaches. We design a plasmonic metalens based on metallic nanorods that, when used with broadband light fields, can beat the diffraction limit for imaging and focusing from the far field. Conventional imaging devices such as optical lenses are limited in resolution by the so-called Rayleigh criterion to half the operating wavelength [1] . Imaging below this resolution requires measuring the evanescent spectrum of an illuminated object, which contains its information on a subwavelength scale, but vanishes exponentially away from it. This can be achieved with near-field scanning optical microscopy (NSOM) [2] , [3] , [4] , but requires point-by-point scanning. The need for real-time super-resolution imaging has led to many proposals of superlenses, high numerical aperture lenses or structured illumination methods [5] , [6] , [7] , [8] , [9] , [10] , [11] , [12] . Those monochromatic approaches, however, still remain limited in resolution, mainly owing to the poor properties of the materials available in the optical range [13] . It was recently demonstrated that an array of subwavelength resonators placed on a subwavelength scale supports wave fields that oscillate on a scale much finer than the free space wavelength due to Fano interferences [14] . Because of the phase shift that the field experiences in the resonator, the spatial scale of the eigenmodes in such an array of resonators is highly frequency dependent around the resonance [14] . Because of their dispersive behaviour, such manmade materials can display very interesting properties when subject to time-dependent wave fields. In fact, shaping the spectrum of a broadband wave impinging on such a medium allows one to control its eigenmodes independently, due to the correspondence of the frequency and spatial dependencies of the wave fields. We have verified experimentally using microwaves [15] and acoustic waves [16] that these wave fields can be efficiently controlled from the far-field and harnessed in order to obtain deep subwavelength focal spots, hence introducing the concept of the resonant metalens. Here we want to prove that a transposition of this concept to the optical domain permits the design of a far-field superlens with unprecedented resolution, even though the materials suffer from high losses in this domain. We show that the use of polychromatic light, which takes advantage of the dispersive properties of optical metamaterials, provides a way to circumvent the limitations associated with monochromatic illumination [17] . We numerically prove that a resonant metalens made out of plasmonic nanoparticles, combined with a femtosecond laser, can potentially focus optical waves onto 30 nm wide foci, λ /23 at the central wavelength of the pulse. We use this lens to demonstrate a real-time far-field imaging scheme based on light pulse echo interferometry, which can image a low-contrast index object with a resolution of 80 nm, which is expected to be improvable. Design of the plasmonic resonant metalens The basis for the plasmonic resonant metalens concept is the design of a medium made of a subwavelength resonant unit cell. Here, we propose to use a metallic nanoparticle to obtain a resonance in the visible range, thanks to the localized plasmon polaritons, but one can also choose to use, for example, a high dielectric nanoparticle as a resonator. To get the smallest resonators possible, we choose a silver nanorod: because of its anisotropy the nanorod presents a resonance along its long axis while its transverse dimension remains much thinner than the free space wavelength. To stay within the limitations of existing fabrication technologies, we set the diameter and height of the nanorod to 30 and 100 nm, respectively, hence keeping an aspect ratio close to three ( Fig. 1a ). We perform three-dimensional simulations of a single nanorod, taking into account losses in silver [18] . As depicted in Fig. 1b , when excited with a plane wave linearly polarized along its long axis, the nanorod exhibits a resonance peak at a wavelength close to 600 nm. 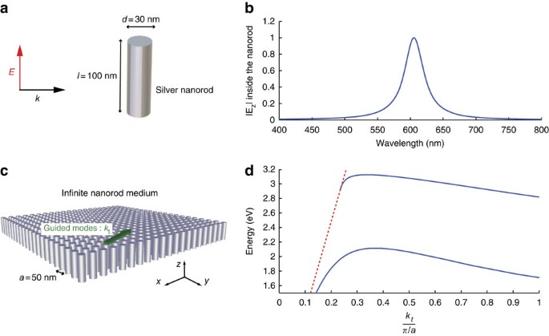Figure 1: The plasmonic resonator-based medium. (a) Geometric parameters of the silver nanorod under the study exhibit a resonance peak around 600 nm (b) when illuminated by light polarized along the rod axis. (c) An infinite medium made of such nanorods organized on a square lattice supports propagating modes along the direction transverse to the rods. Ind, the dispersion relation of the modes (blue curve) shows their subwavelength nature, as the curve is well below the light line (dashed red). Figure 1: The plasmonic resonator-based medium. ( a ) Geometric parameters of the silver nanorod under the study exhibit a resonance peak around 600 nm ( b ) when illuminated by light polarized along the rod axis. ( c ) An infinite medium made of such nanorods organized on a square lattice supports propagating modes along the direction transverse to the rods. In d , the dispersion relation of the modes (blue curve) shows their subwavelength nature, as the curve is well below the light line (dashed red). Full size image To build a resonant metalens, we must create a cluster of such resonators on a subwavelength scale. Here, we choose a square lattice of nanorods with a period of 50 nm, again keeping in mind fabrication feasibility ( Fig. 1c ). Placing these resonant plasmonic nanoparticles on a subwavelength scale induces a strong coupling between them. The medium now supports collective modes with a spatial scale that can be as small as the lattice constant. This strong coupling arises from hybridization between the resonant unit cell and the continuum of free space propagating waves [14] . Such modes are analogous to the nanoparticle chain waveguides [19] , [20] , but in two dimensions. Their dispersion relation is shown in Fig. 1d (see Methods for a detailed description). Because of their subwavelength nature (the dispersion relation is below the light line) the wave fields cannot escape from the top or bottom interfaces and only propagate in the transverse directions. Note that contrary to most of the resonant unit cells, which give rise to a flat dispersion relation at the Brillouin zone's edges and hence to slow light [14] , here an extra near-field coupling that is due to charge accumulations on the sides of the nanorods unfolds this effect. As a consequence, the deep subwavelength modes do not suffer from losses too drastically. Furthermore, the array of nanorods is designed such that the smallest-scale modes, which present the highest wave numbers, appear at a wavelength close to 700 nm, which is the minimum of absorption of silver in the visible range. These two properties are what give our lens its deep subwavelength resolution ability [21] . We now move from the infinite array of resonant nanorods to our far-field superlens, and introduce finiteness along the transverse dimensions. This results in two consequences, which were already described for our microwave resonant metalens [15] , [21] . First, there is a quantization of the eigenmodes supported by the medium. Second, these quantized eigenmodes radiate towards the far-field. To highlight these two facts, we perform a numerical analysis (see Methods) of a 9×9 array of nanorods, which constitutes the resonant metalens ( Fig. 2a ). We first excite the medium with a small dipole source located 25 nm on top of one of the nanorods and polarized along the z axis. This source emits a 5-fs long pulse centred at 700 nm, whose bandwidth covers the entire spectrum of the superlens eigenmodes. As shown in Fig. 2b , the radiated field extends over 200 fs—a consequence of the resonant nature of the medium. This is confirmed by its spectrum that displays many resonant peaks. 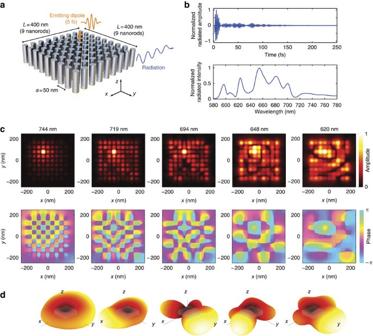Figure 2: Resonant metalens illuminated with polychromatic light. (a) Geometry of the nanorod medium with finite dimensions. When a small dipole placed closed to one nanorod emits a short pulse (5 fs), we measure a radiatedz-polarized electric field in the far-field that extends over 200 fs (b) and exhibits many resonance peaks at distinct frequencies. (c) Amplitude and phase colour maps of the measured near-fields, 25 nm away from the other interface of the medium. Each map shows subwavelength-varying eigenmodes with a spatial scale that strongly depends on the operating frequency. (d) Each of the modes radiates towards the far-field with its own directivity pattern as represented with the isocontour of the radiated intensity. Figure 2: Resonant metalens illuminated with polychromatic light. ( a ) Geometry of the nanorod medium with finite dimensions. When a small dipole placed closed to one nanorod emits a short pulse (5 fs), we measure a radiated z -polarized electric field in the far-field that extends over 200 fs ( b ) and exhibits many resonance peaks at distinct frequencies. ( c ) Amplitude and phase colour maps of the measured near-fields, 25 nm away from the other interface of the medium. Each map shows subwavelength-varying eigenmodes with a spatial scale that strongly depends on the operating frequency. ( d ) Each of the modes radiates towards the far-field with its own directivity pattern as represented with the isocontour of the radiated intensity. Full size image To verify that these peaks correspond to collective eigenmodes of the nanorod medium, we present maps of the near-field of the medium (in amplitude and phase) for various frequencies in Fig. 2c . These maps represent the z -component of the electric field in a plane located 25 nm away from the medium on the side opposite to the source. Each of these near-field maps displays the presence of subwavelength-varying fields with a spatial scale given by the dispersion relation of the infinite medium. This observation proves that the emitting dipole excites the eigenmodes (which do not have a node at the source position) of the medium, and that each frequency corresponds to its own spatial scale thanks to dispersion. The second consequence of the finite dimensions of the medium is the conversion of the subwavelength-varying fields to propagating waves, as already observed when probing the far-field. This conversion owes its efficiency to the resonant nature of the metalens. Now, as each of the modes supported by the medium has its own resonant frequency, their spatial information reaches the far-field as a frequency signature, giving rise to temporal degrees of freedom. The modes have also distinct radiation patterns as shown in Fig. 2d , which this time results in spatial degrees of freedom. It is the conjunction of those spatial and temporal degrees of freedom that give our far-field superlens its unique properties, distinguishing it from monochromatic approaches. Far-field subwavelength focusing of light using time reversal To test the possibilities offered by our lens, we first use it to generate deep subwavelength focal spots from the far-field. To that aim, we use the concept of time-reversal focusing [22] , [23] . This consists of recording the temporal Green's function from a point to a set of detectors, and playing the recorded fields backward in time with the detectors that now act as emitters; it is the polychromatic equivalent of phase conjugation. Very concisely, generating a time-reversed wave field amounts to summing coherently all the modes of a given medium at a specific position with zero relative phase in space and frequency, hence creating a spatio-temporally focused wave field. Following experimental microwaves results [23] , time reversal was used numerically [24] by Li and Stockman to create subwavelength hot spots on random ultra-thin silver films. In our lens, we can engineer which subwavelength modes it supports, and hence focus on any one of the rods. Furthermore, as opposed to the previous transmission scheme [24] , which imposes the use of very thin metallic films, the illumination here is realized azimuthally. In the visible range, there have recently been tremendous achievements in the spatio-temporal control of waves by the use of spatial light modulators (SLMs) and pulse shaping techniques [25] , [26] , [27] , and we believe that the present proposal is experimentally realizable. This supposes, however, that the set of temporal impulse responses between the desired focal position and the set of sources is known. This step is easy to perform numerically but is more challenging experimentally. We propose three different ways to achieve this acquisition. First, one can use a time-resolved NSOM to measure those signals, but this technique may suffer from perturbing effects from the tip. Second, one can imagine exploiting the non-linearity of the silver analogously to what has been done with acoustics waves [28] . One can, for instance, use a SLM as a pulse shaper [25] and maximize the second harmonic generation at a given position on the nanorod array with an adaptive algorithm [28] . This could be realizable from the far-field, as the second harmonic waves are not trapped in the structure (the medium does not support those modes) and a single-focus detection is unlimited in resolution for high enough signal-to-noise ratios. Third, one can characterize the sample with a high-resolution microscope (for example, a scanning electron microscope) and then use a simulation to numerically obtain the experimental signals. Once the impulse response is known, in order to take advantage of the distinct radiation patterns, we emit light from eight distinct directions around the resonant metalens ( Fig. 3a ). Thus, we emit the time-reversed version of the radiated fields in the eight directions when a small dipole, similar to the previous one, emits a short pulse [22] , [23] , [24] . With this method, we obtain a λ /5 (130 nm) spot shown in Fig. 3c , but it is limited to λ /2 by the diffraction limit without the metalens ( Fig. 3b ). Furthermore, because we focus light on a subwavelength scale, an enhancement of the intensity at the focus can be observed. Naturally, we can focus onto each rod by changing the emitted shaped pulses. Shaping the pulse in phase and amplitude, hence, provides even greater flexibility for focusing than polarization-shaping methods [29] . 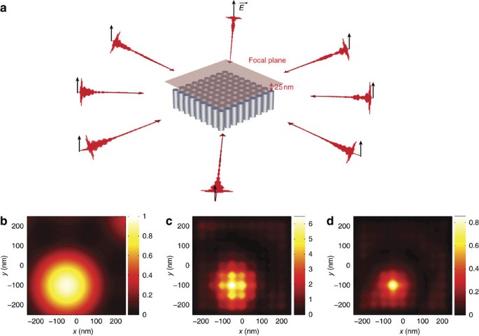Figure 3: Far-field subwavelength focusing. (a) We emit shaped light pulses (that is, time-varying signals) from eight directions in the far-field region and we map the intensity received in the focal plane, 25 nm on top of the nanorods medium. (b) As a control simulation, we show that we obtain an isotropic diffraction-limited focal spot in free space. In the presence of the plasmonic metalens, we obtain (c) aλ/5 wide spot with the emission of signals that correspond to a time-reversal scheme, and (d) aλ/23 wide spot when emitting signals that correspond to an iterative time-reversal scheme. The colour maps are normalized to the emitted energy. Figure 3: Far-field subwavelength focusing. ( a ) We emit shaped light pulses (that is, time-varying signals) from eight directions in the far-field region and we map the intensity received in the focal plane, 25 nm on top of the nanorods medium. ( b ) As a control simulation, we show that we obtain an isotropic diffraction-limited focal spot in free space. In the presence of the plasmonic metalens, we obtain ( c ) a λ /5 wide spot with the emission of signals that correspond to a time-reversal scheme, and ( d ) a λ /23 wide spot when emitting signals that correspond to an iterative time-reversal scheme. The colour maps are normalized to the emitted energy. Full size image Time-reversal focusing has demonstrated its ability to focus on a subwavelength scale from the far-field, but it is not the best candidate in terms of resolution. Indeed, it does not compensate for the relative losses experienced by the modes at distinct frequencies. Much more adequate (in terms of resolution) signals, which behave as spatio-temporal pseudo-inverse filter, can be obtained through an iterative scheme of time reversal [30] . This approach requires the knowledge of the Green's functions between the eight chosen directions and the 81 positions on top of each of the nanorods. Applying this procedure and simulating the whole process, we focus light from the far-field on λ /23 wide spots (30 nm) as shown in Fig. 3d . Again, this is realizable on any rod. Thus, this technique permits one to deposit optical energy on a deep subwavelength scale, from the far-field and dynamically, which could have promising applications in nanolithography or sensing. Polychromatic interferometric far-field subwavelength imaging We have proven that the lens, used with polychromatic light, can focus light from the far-field onto dimensions of the order of 30 nm. This means that it has efficiently projected the deep subwavelength information of the initial source to the far-field. We now use this property to demonstrate that it can also image from the far-field with subwavelength resolution. Again, we assume knowledge of the Green's functions between the eight chosen far-field directions and the 81 nanorods. To verify the possibility of imaging objects with a resolution thinner than the diffraction limit, we place an object in the focal plane of the resonant metalens, that is, 25 nm above it ( Fig. 4a ). The object consists of two dielectric bars with a refractive index of 1.5 and a square cross-section of 30 nm. The distance between the centres of the two objects is 100 nm ( Fig. 4b ). We voluntarily opt for a low-refractive-index-contrast object, which is typical of soft-matter objects. The imaging procedure, described in Fig. 4a , consists solely in far-field operations. Basically, we record the phase and amplitude of the light fields scattered in eight distinct directions when we emit a pulse from one direction. This would experimentally require interferometric measurements. To take advantage of the spatial degrees of freedom offered by our lens, we repeat this operation for the eight directions. Then, from this set of 8×8 temporal signatures that carry the object information, we start the reconstruction of the object. The full description of the imaging procedure is given in the Methods. In Fig. 4b , we map the reconstructed image of the object where each pixel corresponds to a point on top of each nanorod. Meanwhile, we image another object similar to the first one but with one dielectric rod tilted from the main axis of the nanorod array ( Fig. 4c ). To that aim, we use an interpolated set of Green's function (289×8 instead of 81×8). That is, we use the impulse responses between the eight far-field directions and each position of the nanorods and in between nanorods. 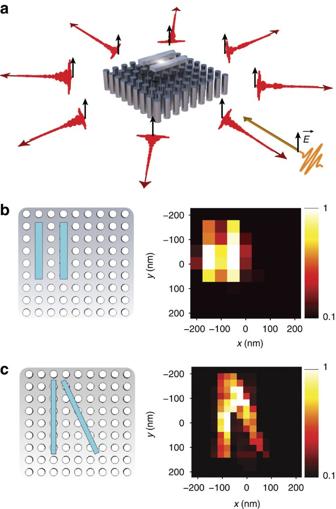Figure 4: Far-field subwavelength imaging of a low contrast object. (a) Acquisition from the far-field of the signals that carry the subwavelength information of the object placed in the near-field of the nanorod medium. We emit a short pulse from one direction (orange line) and receive the time-dependent scattered fields in eight directions (red lines). We repeat this operation for the eight emitting directions. Thebandcpanels show the geometry of an object (left) and the reconstructed super-resolved image from the far-field signals (right). Inb, the distance between the two dielectric bars is 100 nm and the reconstruction clearly shows a resolution of 100 nm. Inc, although the geometry of the object is not entirely aligned along the lattice of the metalens, we still demonstrate a subwavelength-resolved image displaying a 80-nm resolution. Figure 4: Far-field subwavelength imaging of a low contrast object. ( a ) Acquisition from the far-field of the signals that carry the subwavelength information of the object placed in the near-field of the nanorod medium. We emit a short pulse from one direction (orange line) and receive the time-dependent scattered fields in eight directions (red lines). We repeat this operation for the eight emitting directions. The b and c panels show the geometry of an object (left) and the reconstructed super-resolved image from the far-field signals (right). In b , the distance between the two dielectric bars is 100 nm and the reconstruction clearly shows a resolution of 100 nm. In c , although the geometry of the object is not entirely aligned along the lattice of the metalens, we still demonstrate a subwavelength-resolved image displaying a 80-nm resolution. Full size image The image obtained in Fig. 4b clearly shows that the two objects separated by a distance of 100 nm can be resolved from the far-field. Moreover, using the object with a tilted dielectric rod, we verify that an object that is not aligned with the nanorods lattice can be imaged, and we estimate our limiting resolution to about 80 nm. Despite the simplicity of these two objects, those first results prove that the subwavelength information of an object can be registered in the far-field region, thanks to the polychromatic information given by the resonant metalens. Our approach amounts to a parallel and far-field type of NSOM. We underline here that it can be implemented in real time, as it only requires a few illuminations of the sample from the far-field, which can be done using SLMs or movable mirrors. Furthermore, we also mention that although we chose to use only 81 nanorods for computational limitations, it is possible to design much larger lenses while keeping the physics unchanged. This, of course, would result in the presence of much more modes, which in turn would require the control and measurement of the far-field from more directions. The first point we would like to discuss in detail concerns the benefit of using a polychromatic approach and the influence of the spatio-temporal degrees of freedom. Schematically, going from monochromatic to polychromatic waves brings the advantages of frequency modulation over amplitude modulation techniques in radio transmissions. Adopting a polychromatic approach with a resonant metalens multiplies (by the number of independent resonant modes) the degrees of freedom available to the experimentalist for imaging or focusing purposes, compared with the monochromatic case. Here, although the size and properties of the metalens roughly allow the control over eight spatial degrees of freedom, its dispersive nature and the use of polychromatic light increase the degrees of freedom by a factor of approximately ten. These spatio-temporal degrees of freedom can be scrambled by a multiply scattering medium, and hence controlled from the temporal domain, the spatial domain or both [17] . Also, the shape of the metalens, which we chose to be symmetric, could be modified in order to obtain more spatial degrees of freedom; a non-symmetric shape should lift the degeneracy of the modes present in the symmetric metalens, and hence, result in even more degrees of freedom ( Supplementary Fig. S1 ). To underline the importance of the polychromatic approach, we have performed a set of monochromatic-focusing simulations, as well as single-channel time-reversal-focusing simulations. For the monochromatic simulations, we use eight emitting directions and a phase conjugated monochromatic source. For the single channel focusing, we use a single emitting direction but a time-varying optical source. Then, in both cases we probe the intensity in the near-field of the nanorod medium. The monochromatic focal spots obtained for three distinct frequencies ( Fig. 5a ) and the focal spots obtained with one-channel time-reversal simulations for three distinct emitting directions ( Fig. 5b ) both show subwavelength-focusing abilities. Nevertheless, each of these intensity maps present higher side lobes and a wider spot compared with the use of all available spatio-temporal degrees of freedom ( Fig. 3c ). Owing to the recent development of SLMs and pulse-shaping techniques, we therefore insist on the fact that the use of temporal degrees of freedom on top of the spatial ones, that is, the only ones that are usually used with conventional monochromatic schemes, opens many fascinating avenues. 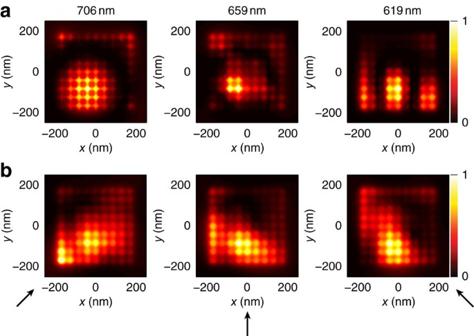Figure 5: Spatio-temporal degrees of freedom. Focal spots obtained when using (a) spatial degrees of freedom only, that is, eight monochromatic sources (at respectively 706 nm, 659 nm and 619 nm), and (b) temporal degrees of freedom only, that is, a single polychromatic source with various angles of incidence (the arrows represent the incident light direction). This underlines the importance of both types of degrees of freedom, as the use of polychromatic and multiple sources gives the thinnest focal spot (Fig. 3c). The color scales are normalized to the focal spot intensity. Figure 5: Spatio-temporal degrees of freedom. Focal spots obtained when using ( a ) spatial degrees of freedom only, that is, eight monochromatic sources (at respectively 706 nm, 659 nm and 619 nm), and ( b ) temporal degrees of freedom only, that is, a single polychromatic source with various angles of incidence (the arrows represent the incident light direction). This underlines the importance of both types of degrees of freedom, as the use of polychromatic and multiple sources gives the thinnest focal spot ( Fig. 3c ). The color scales are normalized to the focal spot intensity. Full size image We also insist on the fact that although we have performed our simulations using optical pulses for simplicity, what really matters for the concept is the polychromatic nature of the light source rather than the duration of the optical wave packets. Both the time-reversal-focusing experiments and the backscattering imaging could be realized using, for instance, supercontinuum sources instead of femtosecond lasers, as both are coherent types of light sources and because we are interested in stationary media. The important point is that the light source should be polychromatic in order to take advantage of all degrees of freedom offered by the metalens, and coherent from one emission to the other. Regarding experimental feasibility, our proposed focusing schemes using time reversal and the emission of eight shaped pulses from eight independent directions may seem rather speculative or experimentally challenging. In fact, such an operation can be drastically simplified without altering its outcome. We have mentioned above that a multiply scattering medium can be used to scramble the spatial and temporal degrees of freedom available to an experimentalist [17] . It is therefore possible to spatio-temporally control a wave field by simply shaping spatially an optical wave front, for instance using a SLM through a thin layer of highly scattering medium [17] , [25] , [26] . If the proposed metalens was sitting on a layer of such a medium, dividing the millions of pixels of a SLM into about 100 macro-pixels should be enough to control the spatio-temporal degrees of freedom of the metalens through it. This type of setup could then be used to focus selectively onto any silver nanorod of the lens using for instance an algorithm, which maximizes the second harmonic generation from silver [28] . Repeating the operation for each rod, one could obtain a complex matrix linking the macro-pixels of the SLM to each nanorod of the medium, and use it for focusing purposes. Of course, the knowledge of this propagation matrix could also be used for the imaging procedure. Although it is fairly impossible to simulate such a setup as a multiply scattering medium consisting of thousands of scattering particles [25] would require gigantic computational resources, this option would nonetheless be the easiest experimental one. Moreover, from an experimental point of view, measurement of noise should be taken into account. There exist several distinct sources of errors during the imaging procedure. First, the imaging is based on an a priori knowledge of a set of far-field Green's functions. Those can be acquired very precisely using many averaging procedures as they have to be obtained only once. Therefore, we will consider that the main source of error during the imaging procedure does not come from the knowledge of those Green's functions. Second, for the image reconstruction, we use signals that are the results of a subtraction. Those subtraction signals present an energy that is six times lower (in average) than the signals before subtraction. However, such an energy ratio does not seem to be limiting with current experimental techniques. The last source of error is the noise during the measurement of the far-field scattered signals. To check the robustness to noise of the imaging procedure, we add numerically a white Gaussian noise to these signals that carry the object information on a subwavelength scale. For distinct levels of noise added to those signals, we run the post-processing steps and reconstruct the image of Fig. 4c . We represent in Fig. 6 the images obtained for four noise levels. When the noise level is below 0.1%, the image obtained is more or less the same as the one obtained without noise ( Fig. 4c ). Increasing the noise level up to 1%, the image is deteriorated but a subwavelength resolution is maintained. Increasing again the noise level, we no longer manage to reconstruct a subwavelength image of the object. Therefore, if we manage to record transient fields with a noise level lower than 1%, the imaging procedure gives a super-resolved image of the object. 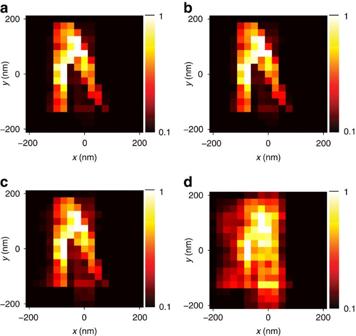Figure 6: Robustness to noise. Ina–d, we add, respectively, 0.01%, 0.1%, 1% and 10% of white noise to the signals received in the far-field before starting the image reconstruction for the object ofFig. 4c. Up to a noise level of 1%, the imaging procedure permits a super-resolved image of the object. Figure 6: Robustness to noise. In a – d , we add, respectively, 0.01%, 0.1%, 1% and 10% of white noise to the signals received in the far-field before starting the image reconstruction for the object of Fig. 4c . Up to a noise level of 1%, the imaging procedure permits a super-resolved image of the object. Full size image Finally, we discuss the imaging resolution of the plasmonic resonant metalens. Because we were able to focus light onto spots as thin as 30 nm from the far-field, one can expect to reach a resolution of 30 nm for the imaging procedure. Indeed, the conversion from evanescent to propagating waves is reciprocal [31] , and as for any lens, the metalens should ultimately present an imaging resolution equal to its focusing resolution. It is clear that the present imaging resolution could be improved by using more sophisticated inversion procedures [32] . Future imaging procedures could also include the modification of the metalens response by the object to image in case of strong interactions, for instance for highly scattering objects such as metallic ones. We also add that, ultimately, the resolution of the proposed metalens is limited by the geometrical parameters one chooses. We have decided to design the metalens such that it is fairly easy to fabricate with existing nano-fabrication technologies, in order to encourage the community to test the proposal experimentally. It is clear, however, that our approach could lead to even smaller focal spots and even better imaging resolutions provided that the spacing between the nanorods as well as their diameter is reduced. This should be realizable, for instance, using aluminium oxyde nanorod templates. In summary, we have proposed to use a medium made of resonant occlusions and to illuminate it with polychromatic light in order to control wave fields on a subwavelength scale from the far-field. We have performed a numerical proof of concept of focusing and imaging below the diffraction limit, from the far-field, with a realistic medium made of silver nanorods. Our approaches are at the frontier of what is achievable with current experimental techniques, but given the incredible recent breakthroughs in the spatio-temporal control of light [33] , we believe that they are experimentally realizable. They could find applications in nanolithography, detection, sensing or subwavelength imaging. Fabry–Perot-based dispersion relation To describe precisely the dispersion law of the propagating waves inside a medium made of nanorods, we can use the recent advances in metamaterials. It has been shown, by the use of an effective medium approach [34] , that an infinite medium made of parallel rods of negative permittivity ɛ supports the propagation of quasi-TEM modes. Those modes propagate at low frequencies [35] , but unlike proper TEM mode at microwaves frequencies, their propagation constant along the rod axis depends on geometry, frequency and transverse wave number k t . In Supplementary Fig. S2 , we plot the theoretical isofrequency curve obtained for our geometry (but with infinite rods) and we superpose the results obtained from two-dimensional simulations with the out-of-plane Comsol RF module solver corresponding to a frequency of 500 THz. This isofrequency curve clearly shows that an infinite medium made of silver rods is spatially dispersive. When adding finiteness along the rods, there is no more effective parameter to describe the medium, but we can give a simple explanation of what happens using the study of the infinite medium [36] . The quasi-TEM mode that exists in the infinite medium travels along the rods and reflects at both interfaces. After a round-trip along the rods this gives rise to a Fabry-Perot resonance. The first Fabry-Perot resonance occurs when the phase shift during a round-trip along the rods equals 2π. This phase shift actually results from two kinds of phase shifts: the first one is due to the propagation along the rods and is given by the isofrequency contours, and the second one ( ϕ ) is due to the reflection at both interfaces. The latter is a well-known phenomenon for total internal reflection and one of its consequences is the Goos–Hanchen shift in the direction transverse to the rods. Therefore, the Fabry–Perot-like resonance manifests itself by a guided propagation along the directions transverse to the nanorods. This happens when the optical path length δ for a round-trip satisfies: where L is the length of the nanorods and n is an integer. From this equation and the phase shift at reflection already calculated [36] , we can write a dispersion relation for the guided waves inside the bounded medium for the first resonance ( n =1): where k is the free space number ( k = ω / c ) and k z is given by the isofrequency contour previously obtained. This implicit theoretical dispersion relation is numerically solved for a matrix of 100 nm long nanorods and plotted in the Fig. 1d . Numerical analysis setup Numerical simulations of the structure were performed using the CST Microwave Studio package with the Transient solver. The nanorod medium consists of an array of 9×9 nanorods made of silver. The behaviour of silver permittivity is obtained with the Johnson and Christy [18] measurements and then interpolated in CST Microwave with a Drude model. The length of the rods L is 100 nm, the period of the lattice a is 50 nm and the diameter of the rods d is 30 nm. The source is a small z- aligned CST discrete port. It is placed at h =25 nm from the top interface of the nanorod medium in the alignment of the fourth nanorod in x and the third one in y -direction. The excitation signal, of duration 5 fs, consists of three sinusoid cycles at 425 THz (symmetric in time), multiplied by a Hanning envelope. Thus, the analysis is performed on a broad range of frequencies from 300 THz up to 700 THz. The background medium, that is, vacuum, extends over 1,400 nm outside the medium in each direction. It is terminated by 'open space' boundary conditions consisting in perfect matched layers with a reflectivity of 10 −6 at 425 THz. We probe the transient electric field in the plane z =125 nm (25 nm away from an interface of the nanorod medium) with a field monitor. The monochromatic near-fields are obtained by Fourier transform in Matlab of the transient recorded near-fields. The far-field is probed with eight CST far-field probes placed at a distance of 1,400 nm outside the medium in the transverse plane that cuts the middle of the rods. In the meantime, we probe the far-field with a broadband far-field monitor in order to obtain the full directivity pattern at each frequency. The transient analysis is stopped when the total simulated time reaches 400 fs. For the focusing scheme, the excitation is performed with plane waves with a k -vector given by the azimuthal angle corresponding to the far-field probe. The emitted signal is the time-reversed version of the signal received by the probe during the first step, and we again probe the transient near-field of the nanorod medium. The result of the eight time-reversal-focusing channels is the summation of the near-field of eight distinct simulations corresponding to eight directions of emission. The focal spots given in Fig. 3b,c correspond to the maximum in time of the squared amplitude of the received signals on each position. The pseudo-inverse-filter signals are obtained in the same way as we have already done in acoustics [16] . We first start by learning the set of 8×81 transient Green's functions, emitting a plane wave from the far-field (and a short pulse) and probing the near-field. Then, we start an iterative procedure [30] that gives us the set of eight signals that focus light on the desired spot. Then we run eight simulations, one for each direction of emissions of the time-varying signal. The focal spot given in Fig. 3d is the summation of the near-field of those eight distinct simulations, as in the time-reversal scheme. All of the focal spots are normalized by the emitted energy. The control experiment gives an intensity of the electric field at the focal position that is, therefore, normalized to unity, as all the frequency components sum constructively (in time and space) at the focal position. When we focus on a thinner scale thanks to the nanorod medium, we measure an electric field intensity at the focal position, which is six times higher than without the nanorods. The pseudo-inverse-filter signals optimize the resolution by increasing the frequency components that suffer from losses. Therefore, this increase of resolution has a cost in terms of deposited energy, and we measure an intensity at the focal position, which is comparable to the one obtained without the nanorods. Imaging procedure The imaging procedure requires the full knowledge of the 8×81 transient impulse responses G ik ( t ) ( i corresponds to the emitting direction and k corresponds to a position on top of one nanorod, that is, a pixel of the image) as stated in the Results. Having knowledge of this bank of data, we run a set of eight simulations, emitting optical pulses from eight distinct directions and recording with far-field probes the signals received in the eight directions, in the presence of the object. We therefore obtain a set of 8×8 temporal signals S ij ( t ) ( i and j correspond, respectively, to the emitting direction and the receiving one). The imaging procedure takes advantage of the subwavelength focusing properties of the resonant metalens. To image the object, the reconstruction procedure numerically focuses onto each rod at emission and reception, as it is often done in ultrasonography. This step is done numerically by convoluting the signals S ij ( t ) and the signals G ik ( -t ) (for focusing at the emission) and then we convolute the result of this operation with G jk ( -t ) again, in order to take advantage of focusing at the reception step. The signal corresponding to the k th pixel of the image is therefore the sum of 8×8 such operations. The pixel's value in the image is the maximum in time of this temporal signal. We repeat those operations for the 81 pixels of the image. The final image is eventually renormalized to have a colour scale varying from 0 to 1. In practice, to increase the resolution of the imaging procedure, we do not use the impulse responses G ik ( t ) for the convolutions, but the signals H ik ( t ) that correspond to the pseudo-inverse-filter signals. That way, we take advantage of the thinnest resolution obtained in the focusing scheme. We also replace the signals S ij ( t ) by the signals S ij ( t )− S 0 ij ( t ), where S 0 ij ( t ) corresponds to the scattered signals in each direction without the object. This way we suppress the diffractive effects coming from the metalens before starting the imaging procedure. How to cite this article: Lemoult, F. et al . A polychromatic approach to far-field superlensing at visible wavelengths. Nat. Commun. 3:889 doi: 10.1038/ncomms1885 (2012).